Loss of NDRG2 expression activates PI3K-AKT signalling via PTEN phosphorylation in ATLL and other cancers Constitutive phosphatidylinositol 3-kinase (PI3K)-AKT activation has a causal role in adult T-cell leukaemia-lymphoma (ATLL) and other cancers. ATLL cells do not harbour genetic alterations in PTEN and PI3KCA but express high levels of PTEN that is highly phosphorylated at its C-terminal tail. Here we report a mechanism for the N-myc downstream-regulated gene 2 (NDRG2)-dependent regulation of PTEN phosphatase activity via the dephosphorylation of PTEN at the Ser380, Thr382 and Thr383 cluster within the C-terminal tail. We show that NDRG2 is a PTEN-binding protein that recruits protein phosphatase 2A (PP2A) to PTEN. The expression of NDRG2 is frequently downregulated in ATLL, resulting in enhanced phosphorylation of PTEN at the Ser380/Thr382/Thr383 cluster and enhanced activation of the PI3K-AKT pathway. Given the high incidence of T-cell lymphoma and other cancers in NDRG2 -deficient mice, PI3K-AKT activation via enhanced PTEN phosphorylation may be critical for the development of cancer. Adult T-cell leukaemia-lymphoma (ATLL) is an aggressive malignant disease of CD4 + T lymphocytes caused by infection with human T-cell leukaemia virus type 1 (HTLV-1) [1] . HTLV-1 is endemic in many regions, including Japan, the Caribbean and parts of South America, and more than 20 million people are infected with this virus worldwide [2] . ATLL develops in ~5% of infected individuals after a long latency period. Although the viral transactivating protein Tax has a crucial role in the proliferation and transformation of the infected T cells, ATLL cells frequently lose their expression of Tax due to genetic and epigenetic changes in the proviral genome [3] . Another viral product, HBZ, has been shown to support the proliferation of ATLL cells; however, additional cellular events are required for the development of ATLL [3] . Recent studies have shown that the phosphatidylinositol 3-kinase (PI3K)-AKT signalling pathway, one of the major oncogenic pathways, is frequently activated in ATLL and is indispensable for the proliferation of ATLL cells [4] , [5] . The phosphatase and tensin homologue (PTEN) deleted on the chromosome 10 ( PTEN ) gene was cloned by association with the human cancer susceptibility locus at 10q23 (refs 6 , 7 ) and is a lipid phosphatase that dephosphorylates phosphatidylinositol 3,4,5-trisphosphate (PIP 3 ) to PI(4,5)P 2 and opposes the PI3K-AKT pathway, exerting tumour suppressor activity [8] . Although PTEN is one of the most frequently mutated genes in human cancer, the frequency of PTEN mutations varies from 1 to 45% [9] . Loss of PTEN through genetic alterations can lead to activation of the AKT pathway; however, activation without PTEN mutations is likely to occur in the majority of cancers, suggesting that different mechanisms such as PIK3CA mutations involve activation of AKT [10] . The lipid phosphatase activity and protein stability of PTEN can be regulated through multiple mechanisms, including acetylation, phosphorylation and ubiquitination [11] . For instance, E3 ubiquitin ligases, NEDD4-1 and WWP2, have been reported to decrease PTEN stability by catalysing PTEN polyubiquitination, and the PTEN degradation predisposes to tumourigenesis [12] , [13] , [14] . In addition, PTEN is subject to phosphorylation at the C-terminal serine–threonine cluster (Ser370, Ser380, Thr382, Thr383 and Ser385) that affects its phosphatase activity, subcellular localization and protein stability [15] , [16] , [17] . It has been proposed that phosphorylation of the C-terminal sites keeps PTEN in an inactive form in the cytoplasm; however, the dephosphorylation induces translocation of PTEN to the plasma membrane where the active PTEN antagonizes PI3K-AKT signalling [18] . PTEN inactivation through increased phosphorylation of the C-terminal serine–threonine cluster is observed in several malignancies, including T-cell acute lymphoblastic leukaemia (T-ALL) [19] , [20] , and casein kinase II (CK2) has been proposed as a candidate protein kinase for the phosphorylation at these sites [21] . However, the molecular mechanisms responsible for this hyperphosphorylation remain poorly understood. Here we identify N-myc downstream-regulated gene 2 (NDRG2) as a PTEN-associated protein that recruits protein phosphatase 2A (PP2A) to facilitate dephosphorylation of PTEN at the Ser380, Thr382 and Thr383 cluster. Our results indicate that genetic and epigenetic inactivation of NDRG2 in ATLL cells leads to increased phosphorylation of PTEN, resulting in decreased PTEN lipid phosphatase activity and subsequent enhanced activation of the PI3K-AKT pathway. Moreover, NDRG2 -deficient mice show high levels of AKT phosphorylation in various tissues and spontaneous tumour development of various types, including T-cell lymphomas, providing the first in vivo evidence that NDRG2 functions as a tumour suppressor gene. Because downregulation of NDRG2 is reported in several types of cancers, the phosphorylation of PTEN at the Ser380/Thr382/Thr383 cluster via NDRG2 inactivation is one of the most important events leading to the dysregulation of PTEN function in cancer. NDRG2 is a candidate tumour suppressor gene in ATLL We recently mapped 605 chromosomal breakpoints in 61 ATLL cases by spectral karyotyping and identified chromosome 14q11 as one of the most common chromosomal breakpoint regions [22] . To map the precise location of the 14q11 chromosomal breakpoints, we performed single-nucleotide polymorphism (SNP)-based comparative genomic hybridization on leukaemia cells from acute-type ATLL patients. In patients with chromosomal deletions at 14q11, the breakpoints frequently accumulated adjacent to the T-cell receptor alpha–delta chain locus (TCRα/δ ), and a recurrent 0.9-Mb interstitial deletion was identified in a region including part of the TCRα/δ locus ( Fig. 1a ). Because tumour suppressors and oncogenes are commonly located at fragile sites [23] , we analysed the expression of the 25 genes that map within the 0.9-Mb region in ATLL cells from seven acute-type ATLL patients and in CD4 + T lymphocytes from the peripheral blood of five healthy volunteers (references) using oligonucleotide microarrays ( Supplementary Methods ) (Affymetrix U133 Plus 2.0). NDRG2 , a member of a new family of differentiation-related genes [24] , and TCR delta variable 3 ( TRDV3 ) were consistently downregulated in all seven ATLL samples compared with the five normal control samples from healthy volunteers ( Fig. 1a ). Furthermore, we used a genome-wide DNA methylation analysis in combination with microarray gene expression analysis to identify genes that are frequently methylated and silenced in ATLL. 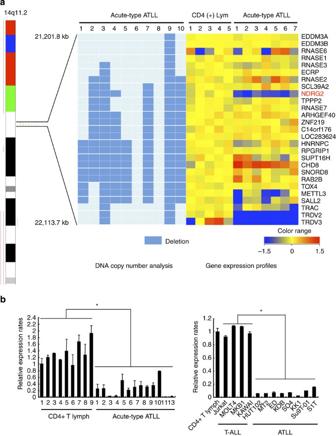Figure 1:NDRG2is a candidate tumour suppressor gene in ATLL. (a) Genomic and gene expression analysis of chromosome 14q11. Results from the SNP array–based comparative genomic hybridization (CGH) analysis on chromosome 14 in ten samples from acute-type ATLL patients. Green bars represent loss of copy number and red bars represent gain of copy number. Out of the ten ATLL samples, eight had breakpoints on 14q11 clustered in a region of 0.9 Mb between genomic positions 21,201,800 and 22,113,700. A heatmap of the normalized gene expression measures for the 27 genes mapped to the recurrent breakpoint region in the CD4+T lymphocytes from five healthy volunteers and ATLL cells from seven acute-type ATLL patients is shown with the deletion map, in which columns represent samples and rows represent genes. A gradient of blue and red colours represent low- and high-relative fold changes of gene expression to the average expression in normal controls. Genes with average signal intensities less than 100 were eliminated. (b) Expression ofNDRG2mRNA in ATLL cells. Quantitative RT–PCR analysis ofNDRG2was performed with mRNA isolated from nine samples of CD4+T lymphocytes from healthy volunteers and 13 samples of ATLL cells from the patients, along with samples from four T-ALL cell lines and eight ATLL cell lines. The relative amounts of mRNA were normalized against β-actin mRNA and expressed relative to the mRNA abundance in healthy control sample 1. Mean±s.d. is shown, *P<0.05 (Mann–WhitneyU-test). More than a 50% reduction inNDRG2mRNA expression was observed in 12 out of 13 cases (92%) of ATLL. Data are representative of two experiments. We identified 34 genes including NDRG2 that become methylated and transcriptionally repressed during ATLL leukaemogenesis ( Supplementary Table 1 , Supplementary Methods ). Here, we investigated whether NDRG2 might be a 14q11 tumour suppressor candidate in ATLL. Quantitative reverse transcription-PCR (RT–PCR) analysis confirmed that NDRG2 expression was significantly reduced in a series of ATLL cell lines and primary acute-type ATLL samples when compared with HTLV-1-negative T-ALL cell lines and CD4 + lymphocytes from healthy volunteers, respectively ( Fig. 1b ). Treatment with an inhibitor of histone deacetylase, trichostatin A, and/or an inhibitor of DNA methylation, 5-aza-deoxycytidine, restored the expression of NDRG2 in most of the ATLL cell lines ( Supplementary Fig. 1 ), suggesting that epigenetic modification is an important mechanism to reduce the expression of NDRG2 in ATLL cells. In accordance with DNA methylation array data, the CpG islands of the NDRG2 promoter were heavily methylated in three ATLL cell lines and primary ATLL cells from five acute-type ATLL patients, but not in three T-ALL cell lines and control CD4 + lymphocytes from five healthy volunteers, as revealed by bisulfite-sequencing analysis ( Supplementary Fig. 2 ). 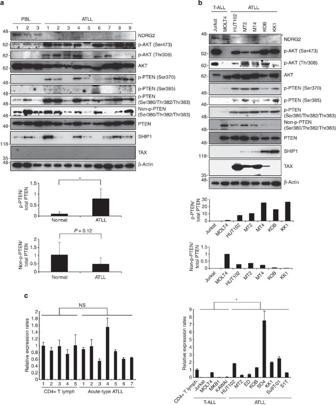Figure 2: The PI3K-AKT signalling pathway is activated in ATLL cells. (a) A western blot analysis of NDRG2, PTEN, phosphorylated PTEN (p-PTEN) (Ser370, Ser380/Thr382/Thr383 and Ser385), non-p-PTEN (Ser380/Thr382/Thr383), SHIP1, AKT, p-AKT (Ser473 and Thr308) and Tax was performed in primary leukaemic cells from acute-type ATLL patients. The CD4+T lymphocytes from healthy volunteers (CD4+T lymph) served as the controls. No expression of Tax was detected in CD4+T lymphocytes from healthy volunteers or ATLL cells from acute-type ATLL patients. The graph shows relative band intensity of p-PTEN (Ser380/Thr382/Thr383) and non-p-PTEN (Ser380/Thr382/Thr383). Each p-PTEN or non-p-PTEN value was divided by the total PTEN value for a given sample. The data are expressed as the mean value±s.d. (*P<0.05, Student’st-test). The data are representative of three experiments. (b) A western blot analysis with the same antibodies as inFig. 2awas performed in the T-ALL and ATLL cell lines. Asterisk, nonspecific band. HTLV-1-transformed T-cell lines (HUT102, MT2 and MT4) expressed high levels of Tax. The graph shows relative band intensity of p-PTEN (Ser380/Thr382/Thr383) and non-p-PTEN (Ser380/Thr382/Thr383). Each p-PTEN or non-p-PTEN value was divided by the total PTEN value for a given sample. The data are representative of three experiments. (c) Quantitative RT–PCR analysis ofPTENin CD4+T lymphocytes from five healthy volunteers and ATLL cells from seven acute-type ATLL patients, along with four T-ALL cell lines and eight ATLL cell lines. The relative amounts of mRNA were normalized against β-actin mRNA and expressed relative to the mRNA abundance in healthy control sample 1. The mean±s.d. is shown; *P<0.05; NS, not significant (Mann–WhitneyU-test). The data are representative of two experiments. Similarly, a methylation-specific PCR confirmed the hypermethylation of the NDRG2 promoter in the majority of ATLL cells (eight of eight ATLL cell lines and 34 of 34 primary samples) ( Supplementary Table 2 ). 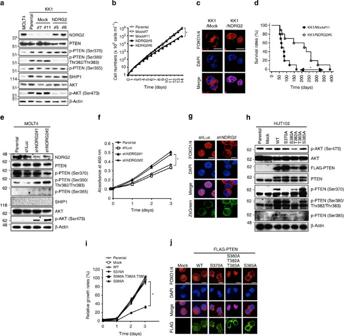Figure 3: Decreased expression ofNDRG2and the enhanced phosphorylation of PTEN are involved in the activation of PI3K-AKT. (a) Western blots analysis of stably transfected KK1 cells. Note that the amount of NDRG2 protein in both MOLT4 and NDRG2-transfected KK1 cells was found to be similar. The data are representative of three experiments. (b) The proliferation rates of KK1-NDRG2, KK1-Mock, and parental KK1 cells. The mean±s.d. is shown; *P<0.05 (Student’st-test). The data are representative of three experiments. (c) The subcellular localization of FOXO1/4 in KK1-NDRG2 and KK1-Mock cells. The nuclei were labelled with DAPI. Scale bar, 10 μm. The data are representative of three experiments. (d) Kaplan–Meier survival curves of NOG mice intravenously injected with KK1-NDRG2 or KK1-Mock cells (n=10 mice per group, *P<0.05, log-rank test). (e) MOLT4 cells transiently transfected with two different shRNAs against NDRG2 or control shRNA against luciferase (shLuc) were subjected to western blotting. The data are representative of three experiments. (f) The proliferation rates of MOLT4 cells transfected with shNDRG2 or shLuc expression vectors. The mean±s.d. is shown; *P<0.05 (Student’st-test). The data are representative of three experiments. (g) The subcellular localization of FOXO1/4 in MOLT4 cells transfected with shNDRG2 or shLuc. The transfected cells were visualized by ZsGreen expression. Scale bar, 10 μm. The data are representative of three experiments. (h) HUT102 cells transfected with WT PTEN or PTEN mutants were subjected to western blotting. A slower migrating band for PTEN and phosphorylated PTEN appears in the presence of transfected PTEN, and a high level of phosphorylation of exogenous PTEN-Ser380/Thr382/Thr383 was observed in HUT102 cells. The data are representative of three experiments. (i) The proliferation rates of HUT102 cells transfected with WT or mutant PTEN. The mean±s.d. is shown; *P<0.05 (Student’st-test). The data are representative of three experiments. (j) The subcellular localization of FOXO1/4 in HUT102 cells transfected with WT or mutant PTEN. The transfected cells were visualized using an antibody against FLAG. Scale bar, 10 μm. The data are representative of three experiments. 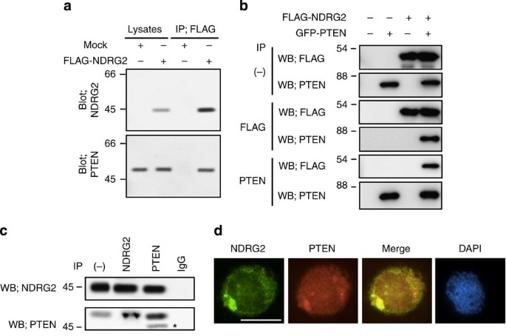Figure 4: NDRG2 is a novel PTEN-interacting protein. (a) The KK1 cell lysates transfected with the mock or FLAG-NDRG2 vector were immunoprecipitated with an anti-FLAG antibody, and the western blots were probed with the indicated antibodies. IP, immunoprecipitation. The data are representative of three experiments. (b) Exogenously expressed PTEN and NDRG2 were co-immunoprecipitated in 293T cells (WB, western blot). The data are representative of three experiments. (c) The co-immunoprecipitation of endogenous PTEN and NDRG2 was performed in MOLT4 cell lysates. On the input lane (−), 1/200 of the input was loaded for detection of NDRG2. Asterisk, nonspecific band. The data are representative of three experiments. (d) The co-localization of endogenous PTEN and NDRG2 was determined in MOLT4 cells. The nuclei were labelled with DAPI. Scale bar, 10 μm. The data are representative of three experiments. No somatic mutations in the NDRG2 gene were observed in 34 primary ATLL samples and 42 cancer cell lines, including eight ATLL cell lines ( Supplementary Table 3 ), except for previously reported SNPs ( Supplementary Table 4 ). These data indicated that NDRG2 is frequently inactivated by genomic deletion and epigenetic silencing in ATLL. Figure 1: NDRG2 is a candidate tumour suppressor gene in ATLL. ( a ) Genomic and gene expression analysis of chromosome 14q11. Results from the SNP array–based comparative genomic hybridization (CGH) analysis on chromosome 14 in ten samples from acute-type ATLL patients. Green bars represent loss of copy number and red bars represent gain of copy number. Out of the ten ATLL samples, eight had breakpoints on 14q11 clustered in a region of 0.9 Mb between genomic positions 21,201,800 and 22,113,700. A heatmap of the normalized gene expression measures for the 27 genes mapped to the recurrent breakpoint region in the CD4 + T lymphocytes from five healthy volunteers and ATLL cells from seven acute-type ATLL patients is shown with the deletion map, in which columns represent samples and rows represent genes. A gradient of blue and red colours represent low- and high-relative fold changes of gene expression to the average expression in normal controls. Genes with average signal intensities less than 100 were eliminated. ( b ) Expression of NDRG2 mRNA in ATLL cells. Quantitative RT–PCR analysis of NDRG2 was performed with mRNA isolated from nine samples of CD4 + T lymphocytes from healthy volunteers and 13 samples of ATLL cells from the patients, along with samples from four T-ALL cell lines and eight ATLL cell lines. The relative amounts of mRNA were normalized against β-actin mRNA and expressed relative to the mRNA abundance in healthy control sample 1. Mean±s.d. is shown, * P <0.05 (Mann–Whitney U -test). More than a 50% reduction in NDRG2 mRNA expression was observed in 12 out of 13 cases (92%) of ATLL. Data are representative of two experiments. Full size image The PI3K-AKT signalling pathway is activated in ATLL cells Because the PI3K-AKT signalling pathway is constitutively activated in ATLL cells [4] , we analysed PTEN and NDRG2 expression and the activation status of PI3K-AKT in primary ATLL cells from acute-type ATLL patients and in ATLL cell lines ( Fig. 2a,b ). The NDRG2 protein expression in ATLL cell lines and primary ATLL cells was significantly lower than that in T-ALL cell lines and CD4 + lymphocytes from healthy volunteers, and AKT phosphorylation at Ser473 and Thr308, an indicator of AKT activation, was detected in the majority of the primary ATLL samples and ATLL cell lines. Because PTEN mRNA and protein were expressed at normal levels in all of the ATLL samples except the SO4 cell line ( Fig. 2c ), we performed a mutation analysis of the PTEN and PIK3CA genes. No mutations were detected within the coding and adjacent intronic regions of PTEN or in the hotspot mutation regions of PIK3CA in the ATLL samples ( Supplementary Table 3 ). Therefore, we considered the possibility that post-translational modifications of PTEN influence PTEN phosphatase activity in ATLL cells. The phosphorylation of PTEN at the serine–threonine cluster (Ser370, Ser380, Thr382, Thr383 and Ser385) in the C-terminal tail suppresses its phosphatase activity [17] ; therefore, we evaluated PTEN phosphorylation and demonstrated that the cluster sites were highly phosphorylated in the primary ATLL cells and ATLL cell lines, whereas the non-phosphorylated form was lower in abundance compared with controls ( Fig. 2a,b ; Supplementary Fig. 3 ). Notably, we also found that the SO4 cell line, which has a higher level of PTEN expression, contains high levels of phosphorylated PTEN and an elevated level of phosphorylated AKT ( Supplementary Fig. 4 ). Furthermore, the expression levels of SHIP1, a different class of lipid phosphatase that catalyses PIP 3 to PI(3,4)P 2 (ref. 25 ), showed no significant differences between ATLL cells and controls, although a few cases showed higher levels of SHIP1 ( Fig. 2a,b ). Collectively, these results suggested that PI3K-AKT pathway activation in ATLL may be related to increased PTEN phosphorylation and potentially to the inactivation of NDRG2 . Figure 2: The PI3K-AKT signalling pathway is activated in ATLL cells. ( a ) A western blot analysis of NDRG2, PTEN, phosphorylated PTEN (p-PTEN) (Ser370, Ser380/Thr382/Thr383 and Ser385), non-p-PTEN (Ser380/Thr382/Thr383), SHIP1, AKT, p-AKT (Ser473 and Thr308) and Tax was performed in primary leukaemic cells from acute-type ATLL patients. The CD4 + T lymphocytes from healthy volunteers (CD4 + T lymph) served as the controls. No expression of Tax was detected in CD4 + T lymphocytes from healthy volunteers or ATLL cells from acute-type ATLL patients. The graph shows relative band intensity of p-PTEN (Ser380/Thr382/Thr383) and non-p-PTEN (Ser380/Thr382/Thr383). Each p-PTEN or non-p-PTEN value was divided by the total PTEN value for a given sample. The data are expressed as the mean value±s.d. (* P <0.05, Student’s t- test). The data are representative of three experiments. ( b ) A western blot analysis with the same antibodies as in Fig. 2a was performed in the T-ALL and ATLL cell lines. Asterisk, nonspecific band. HTLV-1-transformed T-cell lines (HUT102, MT2 and MT4) expressed high levels of Tax. The graph shows relative band intensity of p-PTEN (Ser380/Thr382/Thr383) and non-p-PTEN (Ser380/Thr382/Thr383). Each p-PTEN or non-p-PTEN value was divided by the total PTEN value for a given sample. The data are representative of three experiments. ( c ) Quantitative RT–PCR analysis of PTEN in CD4 + T lymphocytes from five healthy volunteers and ATLL cells from seven acute-type ATLL patients, along with four T-ALL cell lines and eight ATLL cell lines. The relative amounts of mRNA were normalized against β-actin mRNA and expressed relative to the mRNA abundance in healthy control sample 1. The mean±s.d. is shown; * P <0.05; NS, not significant (Mann–Whitney U -test). The data are representative of two experiments. Full size image NDRG2 expression induces dephosphorylation of PTEN and AKT To determine whether low NDRG2 expression was associated with increased PTEN phosphorylation and PI3K-AKT activation in ATLL cells, we introduced an NDRG2 expression vector into two ATLL cell lines (KK1 and HUT102). The phosphorylation of AKT-Ser473 and PTEN-Ser380/Thr382/Thr383, but not PTEN-Ser370 and PTEN-Ser385, was markedly decreased in both NDRG2-expressing cell lines ( Fig. 3a ; Supplementary Fig. 5a ), although NDRG2 expression did not significantly change the basal activity of PI3K ( Supplementary Fig. 6 ). There was also an increase in the abundance of Ser380/Thr382/Thr383 non-phosphorylated PTEN in NDRG2-expressing cells ( Supplementary Fig. 7 ). No change in SHIP1 expression was detected ( Fig. 3a ). In addition, the NDRG2-transfected cells exhibited decreased growth rates and a predominant nuclear localization of forkhead box protein O1 and O4 (FOXO1/4) (a marker of low AKT activity status) ( Fig. 3b,c ; Supplementary Fig. 5b ). Furthermore, to determine whether NDRG2 expression may influence the tumour growth of transplanted ATLL cells in vivo , mock vector-transfected or NDRG2-transfected KK1 cells were injected intravenously into NOD/Shi- scid , interleukin (IL)-2Rg null (NOG) mice. The average duration of life of 10 mice after inoculation with KK1-Mock cells was 67 days, but that of 10 mice inoculated with KK1-NDRG2 cells was extended to 207 days ( Fig. 3d ; Supplementary Fig. 8 ). Statistically significant difference in apoptotic cell rate was also found in the infiltrating neoplastic cells between KK1-Mock- and KK1-NDRG2-injected mice ( Supplementary Fig. 9 ). To investigate these observations further, we performed the reverse experiment by inhibiting NDRG2 expression in the MOLT4 cell line. Transfection of the MOLT4 cell line with short hairpin RNA (shRNA) against NDRG2 enhanced the phosphorylation of PTEN-Ser380/Thr382/Thr383 and AKT-Ser473, which was accompanied by increased cell proliferation and a relocation of FOXO1/4 from the nucleus to the cytoplasm ( Fig. 3e–g ). We utilized the NIH3T3 mouse embryonic fibroblast cell line to confirm whether NDRG2 expression attenuates PTEN-Ser380/Thr382/Thr383 phosphorylation and AKT activation. After serum stimulation or transfection of a constitutively active PI3K mutant, we determined that the inhibition of NDRG2 expression resulted in increases in phosphorylated PTEN-Ser380/Thr382/Thr383 and AKT-Ser473 compared with the control cells ( Supplementary Figs 10 and 11 ). In contrast, the forced expression of NDRG2 in NIH3T3 cells resulted in a dose-dependent decrease in PTEN-Ser380/Thr382/Thr383 and AKT-Ser473 phosphorylation under conventional culture conditions ( Supplementary Fig. 12 ). To establish a direct link between PTEN-Ser380/Thr382/Thr383 phosphorylation and PI3K-AKT activation, we constructed PTEN-S370A, -S380A/T382A/T383A and -S385A mutants in which Ser370, a Ser380/Thr382/Thr383 cluster and Ser385, respectively, were replaced with alanines. The forced expression of the PTEN-S380A/T382A/T383A mutant in HUT102 cells decreased AKT phosphorylation, cell growth and nuclear localization of FOXO1/4, whereas the expression of the PTEN-S370A or PTEN-S385A mutant had no significant effect ( Fig. 3h–j ). Treatment of ATLL cells with the CK2 inhibitors, 4,5,6,7-tetrabromobenzotriazole (TBB) and CX-4945, did not change the level of phosphorylated PTEN-Ser380/Thr382/Thr383, whereas the same treatment decreased PTEN-Ser370, a bona fide CK2 substrate [26] , and AKT-Ser473 phosphorylation ( Supplementary Fig. 13 ). These results indicate that the phosphorylation on PTEN-Ser380/Thr382/Thr383 has an important role in the activation of PI3K-AKT in ATLL cells, and that NDRG2 is able to reverse PTEN-Ser380/Thr382/Thr383 phosphorylation, leading to the suppression of PI3K-AKT activation. Figure 3: Decreased expression of NDRG2 and the enhanced phosphorylation of PTEN are involved in the activation of PI3K-AKT. ( a ) Western blots analysis of stably transfected KK1 cells. Note that the amount of NDRG2 protein in both MOLT4 and NDRG2-transfected KK1 cells was found to be similar. The data are representative of three experiments. ( b ) The proliferation rates of KK1-NDRG2, KK1-Mock, and parental KK1 cells. The mean±s.d. is shown; * P <0.05 (Student’s t- test). The data are representative of three experiments. ( c ) The subcellular localization of FOXO1/4 in KK1-NDRG2 and KK1-Mock cells. The nuclei were labelled with DAPI. Scale bar, 10 μm. The data are representative of three experiments. ( d ) Kaplan–Meier survival curves of NOG mice intravenously injected with KK1-NDRG2 or KK1-Mock cells ( n =10 mice per group, * P <0.05, log-rank test). ( e ) MOLT4 cells transiently transfected with two different shRNAs against NDRG2 or control shRNA against luciferase (shLuc) were subjected to western blotting. The data are representative of three experiments. ( f ) The proliferation rates of MOLT4 cells transfected with shNDRG2 or shLuc expression vectors. The mean±s.d. is shown; * P <0.05 (Student’s t- test). The data are representative of three experiments. ( g ) The subcellular localization of FOXO1/4 in MOLT4 cells transfected with shNDRG2 or shLuc. The transfected cells were visualized by ZsGreen expression. Scale bar, 10 μm. The data are representative of three experiments. ( h ) HUT102 cells transfected with WT PTEN or PTEN mutants were subjected to western blotting. A slower migrating band for PTEN and phosphorylated PTEN appears in the presence of transfected PTEN, and a high level of phosphorylation of exogenous PTEN-Ser380/Thr382/Thr383 was observed in HUT102 cells. The data are representative of three experiments. ( i ) The proliferation rates of HUT102 cells transfected with WT or mutant PTEN. The mean±s.d. is shown; * P <0.05 (Student’s t- test). The data are representative of three experiments. ( j ) The subcellular localization of FOXO1/4 in HUT102 cells transfected with WT or mutant PTEN. The transfected cells were visualized using an antibody against FLAG. Scale bar, 10 μm. The data are representative of three experiments. Full size image NDRG2 is a novel PTEN-interacting protein To determine whether NDRG2 physically associates with PTEN, lysates from KK1 cells stably expressing FLAG-tagged NDRG2 were immunoprecipitated with an anti-FLAG antibody, and NDRG2-associated proteins were analysed by western blotting with a PTEN-specific antibody. We found that ectopically expressed NDRG2 co-precipitated with endogenous PTEN in ATLL cells ( Fig. 4a ). Exogenously expressed green fluorescent protein (GFP)-tagged PTEN and FLAG-tagged NDRG2 co-precipitated in 293T cells ( Fig. 4b ), and endogenous NDRG2 and PTEN co-immunoprecipitated with each specific antibody and co-localized in the cytoplasm in MOLT4 cells ( Fig. 4c,d ), suggesting that these two proteins physically interact in T lymphocytes. By subjecting a series of deletion mutants to co-immunoprecipitation assays, a domain containing a putative α–β hydrolase fold (NDR domain) that is conserved among NDRG family members [27] was found to interact with the C-terminal half of PTEN, which contains a C2 lipid-binding domain ( Supplementary Fig. 14 ). In addition, the S370A, S380A/T382A/T383A and S385A mutations in PTEN did not significantly interfere with the binding of NDRG2 ( Supplementary Fig. 15 ), suggesting that NDRG2 can bind to both the phosphorylated and non-phosphorylated forms of PTEN. Figure 4: NDRG2 is a novel PTEN-interacting protein. ( a ) The KK1 cell lysates transfected with the mock or FLAG-NDRG2 vector were immunoprecipitated with an anti-FLAG antibody, and the western blots were probed with the indicated antibodies. IP, immunoprecipitation. The data are representative of three experiments. ( b ) Exogenously expressed PTEN and NDRG2 were co-immunoprecipitated in 293T cells (WB, western blot). The data are representative of three experiments. ( c ) The co-immunoprecipitation of endogenous PTEN and NDRG2 was performed in MOLT4 cell lysates. On the input lane (−), 1/200 of the input was loaded for detection of NDRG2. Asterisk, nonspecific band. The data are representative of three experiments. ( d ) The co-localization of endogenous PTEN and NDRG2 was determined in MOLT4 cells. The nuclei were labelled with DAPI. Scale bar, 10 μm. The data are representative of three experiments. Full size image NDRG2 recruits PP2A to dephosphorylate PTEN To determine the mechanism by which NDRG2 expression induces PTEN dephosphorylation, we incubated KK1-NDRG2 cell lysates with a synthetic PTEN phosphopeptide containing the Ser380/Thr382/Thr383 cluster in the presence or absence of increasing concentrations of okadaic acid (OA), an inhibitor of the serine–threonine phosphatases, PP1 and PP2A [28] . We incubated KK1/NDRG2 cell lysates with the synthetic pSer380/pThr382/pThr383 peptide in the presence or absence of increasing concentrations of OA. As expected, the phosphatase activity in KK1-NDRG2 cell lysates was substantially inhibited by a low concentration of OA (10 nM) ( Fig. 5a ). In addition, the dephosphorylation of PTEN-Ser380/Thr382/Thr383 in KK1-NDRG2 cells was inhibited by OA in a dose-dependent manner ( Fig. 5b ), but there was no effect on PTEN-Ser370 phosphorylation. In accordance with these results, a transiently expressed PP2A catalytic subunit (PP2Ac), but not PP1c or PP5c, efficiently dephosphorylated the synthetic pSer380/pThr382/pThr383 peptide, which was prevented by 10 nM OA ( Fig. 5c ; Supplementary Fig. 16 ). Similarly, the endogenous PP2Ac immunoprecipitated from NIH3T3 lysates exhibited phosphatase activity toward the pSer380/pThr382/pThr383 peptide in an OA-sensitive manner ( Fig. 5d ; Supplementary Fig. 17 ). In support of these data, small interfering RNA (siRNA)-mediated knockdown of PP2Acα prevented the NDRG2-dependent PTEN dephosphorylation in KK1-NDRG2 cells ( Supplementary Fig. 18 ). Further analysis revealed that the recombinant PP2A core enzyme, a dimer of PP2Ac and the structural A subunit, also dephosphorylated the pSer380/pThr382/pThr383 peptide and was capable of dephosphorylating each of the three phosphorylated residues (pSer380, pThr382 and pThr383) with comparable efficiencies ( Fig. 5e ). Recombinant PP2A dephosphorylated PTEN-Ser380/Thr382/Thr383 purified from KK1 cell lysates ( Fig. 5f ), indicating that PP2A specifically mediates the dephosphorylation of PTEN-Ser380/Thr382/Thr383. We demonstrated that PP2Ac co-precipitated with NDRG2 in the lysates of crosslinked HUT102/NDRG2 cells ( Fig. 5g ). Although PP2Ac was barely detectable in the PTEN immunoprecipitates from KK1-Mock cells ( Fig. 5h ), PTEN clearly co-precipitated with both NDRG2 and PP2Ac in KK1-NDRG2 cells; this result was accompanied by decreased PTEN-Ser380/Thr382/Thr383 phosphorylation ( Fig. 5h ), suggesting that NDRG2 recruits PP2A to PTEN and thereby promotes PTEN-Ser380/Thr382/Thr383 dephosphorylation. Remarkably, we found that C-terminal deletion mutants of NDRG2 (ΔC and NDR), which do not interact with PP2A, are impaired in their ability to downregulate PTEN-Ser380/Thr382/Thr383 phosphorylation ( Supplementary Fig. 19 ). 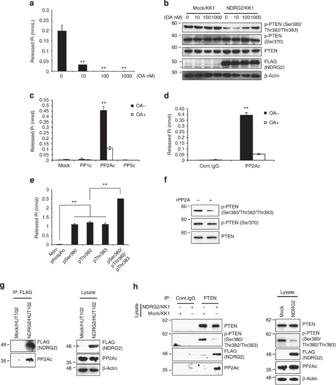Figure 5: NDRG2 recruits PP2A to PTEN leading to its dephosphorylation at pSer380/pThr382/pThr383. (a) KK1-NDRG2 cell lysates were incubated with a pSer380/pThr382/pThr383 PTEN phosphopeptide in the presence or absence of different concentrations of OA. The amount of released phosphate was quantitated using the malachite green assay. The mean±s.d. is shown; **P<0.05 compared with untreated control (Student’st-test). The data are representative of three experiments. (b) KK1-Mock and KK1-NDRG2 cells were treated with increasing concentrations of OA for 2 h and subjected to western blot analysis. Asterisk, nonspecific band. The data are representative of three experiments. (c) After immunoprecipitating lysates from 293T cells transfected with the indicated vectors, the beads were incubated with a pSer380/pThr382/pThr383 phosphopeptide in the presence or absence of 10 nM OA, and phosphate release was determined. The mean±s.d. is shown; **P<0.05 (Student’st-test). The data are representative of three experiments. (d) After immunoprecipitating the NIH3T3 lysates with an anti-PP2Ac antibody, the beads were incubated with a pSer380/pThr382/pThr383 phosphopeptide in the presence or absence of 10 nM OA, and phosphate release was determined. The mean±s.d. is shown; **P<0.05 (Student’st-test). The data are representative of three experiments. (e) 0.5 unit of recombinant PP2A was incubated with 200 μg ml−1of either PTEN peptide or the phosphopeptides containing either pSer380, pThr382, pThr383 or pSer380/pThr382/pThr383, and phosphate release was determined. The mean±s.d. is shown; **P<0.05 (Student’st-test). The data are representative of three experiments. (f) The beads were incubated with or without recombinant PP2A after immunoprecipitating the KK1-Mock lysates with an anti-PTEN antibody. Western blot analysis of the reaction mixtures was performed to determine the degree of phosphorylation of PTEN. The data are representative of two experiments. (g) The lysates of HUT102-NDRG2 or HUT102-Mock cells treated with the crosslinker DTBP were immunoprecipitated with an anti-FLAG antibody and subsequently probed for co-precipitated PP2Ac by Western blotting. The data are representative of three experiments. (h) The lysates from KK1-NDRG2 or KK1-Mock cells treated with DTBP were immunoprecipitated with an anti-PTEN antibody, and the Western blots were probed with the indicated antibodies. Asterisk, nonspecific band. The data are representative of three experiments. Figure 5: NDRG2 recruits PP2A to PTEN leading to its dephosphorylation at pSer380/pThr382/pThr383. ( a ) KK1-NDRG2 cell lysates were incubated with a pSer380/pThr382/pThr383 PTEN phosphopeptide in the presence or absence of different concentrations of OA. The amount of released phosphate was quantitated using the malachite green assay. The mean±s.d. is shown; ** P <0.05 compared with untreated control (Student’s t- test). The data are representative of three experiments. ( b ) KK1-Mock and KK1-NDRG2 cells were treated with increasing concentrations of OA for 2 h and subjected to western blot analysis. Asterisk, nonspecific band. The data are representative of three experiments. ( c ) After immunoprecipitating lysates from 293T cells transfected with the indicated vectors, the beads were incubated with a pSer380/pThr382/pThr383 phosphopeptide in the presence or absence of 10 nM OA, and phosphate release was determined. The mean±s.d. is shown; ** P <0.05 (Student’s t- test). The data are representative of three experiments. ( d ) After immunoprecipitating the NIH3T3 lysates with an anti-PP2Ac antibody, the beads were incubated with a pSer380/pThr382/pThr383 phosphopeptide in the presence or absence of 10 nM OA, and phosphate release was determined. The mean±s.d. is shown; ** P <0.05 (Student’s t- test). The data are representative of three experiments. ( e ) 0.5 unit of recombinant PP2A was incubated with 200 μg ml −1 of either PTEN peptide or the phosphopeptides containing either pSer380, pThr382, pThr383 or pSer380/pThr382/pThr383, and phosphate release was determined. The mean±s.d. is shown; ** P <0.05 (Student’s t- test). The data are representative of three experiments. ( f ) The beads were incubated with or without recombinant PP2A after immunoprecipitating the KK1-Mock lysates with an anti-PTEN antibody. Western blot analysis of the reaction mixtures was performed to determine the degree of phosphorylation of PTEN. The data are representative of two experiments. ( g ) The lysates of HUT102-NDRG2 or HUT102-Mock cells treated with the crosslinker DTBP were immunoprecipitated with an anti-FLAG antibody and subsequently probed for co-precipitated PP2Ac by Western blotting. The data are representative of three experiments. ( h ) The lysates from KK1-NDRG2 or KK1-Mock cells treated with DTBP were immunoprecipitated with an anti-PTEN antibody, and the Western blots were probed with the indicated antibodies. Asterisk, nonspecific band. The data are representative of three experiments. Full size image NDRG2 -deficient mice are susceptible to spontaneous tumours To determine whether NDRG2 has a role in tumourigenesis, we generated NDRG2 -deficient ( NDRG2 −/− ) mice ( Supplementary Fig. 20 ), which were born at normal Mendelian ratios ( Supplementary Table 5 ) and developed without apparent physical abnormalities. NDRG2 was highly expressed in the adult mouse brain, heart and liver [29] ( Fig. 6a ). The mutant mice exhibited increased levels of phosphorylated PTEN-Ser380/Thr382/Thr383, AKT-Ser473 and GSK3β-Ser9 in all of the tissues examined ( Fig. 6b ). In addition to the NDRG2 and PTEN interaction in the frontal cortex of wild-type (WT) mice ( Fig. 6c ), the NDRG2 −/− embryonic fibroblasts exhibited increased phosphorylated PTEN-Ser380/Thr382/Thr383, high AKT-Ser473 phosphorylation and an accelerated cell proliferation rate ( Fig. 6d,e ). The NDRG2 −/− mice had a markedly shorter lifespan than the WT or NDRG2 +/− mice ( Fig. 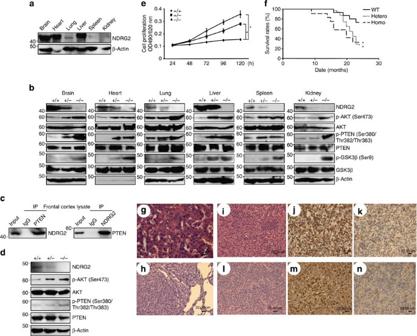Figure 6:NDRG2-deficient mice are susceptible to tumour formation. (a) Western blots of 3-month-old adult tissues of WT mice. The data are representative of two experiments. (b) Western blots of various tissues of 3-month-oldNDRG2-deficient mice. The data are representative of two experiments. (c) The co-immunoprecipitation of PTEN and NDRG2 in frontal cortex homogenates from 3-month-old WT mice. The data are representative of three experiments. (d) Whole-cell lysates from WT,NDRG2+/−andNDRG2−/−embryonic fibroblasts were subjected to western blotting. (e) The proliferation rates of WT,NDRG2+/−, andNDRG2−/−embryonic fibroblasts. The mean±s.d. is shown; *P<0.05 (Student’st-test). The data are representative of three experiments. (f) Kaplan–Meier survival curves of WT (n=15),NDRG2+/−(n=31) andNDRG2−/−(n=12) mice up to 24 months of age. The difference in survival was statistically significant between WT andNDRG2+/−orNDRG2−/−mice (*P<0.05, log-rank test). (g) A hepatocellular carcinoma section from anNDRG2+/−mouse liver was subjected to H&E staining. The results indicated the presence of a large sheet of hepatic cords composed of several hepatocytes of variable nuclei and cell sizes; the nuclei of the carcinoma cells were hyperchromatic with prominent nucleoli (scale bar, 22 μm). (h) A bronchoalveolar carcinoma section from anNDRG2+/−mouse lung was subjected to H&E staining. The histopathology demonstrated a well-circumscribed mass of a solid sheet of neoplastic cells containing hyperchromatic nuclei with signs of frequent mitosis and an indistinct basophilic cytoplasm (scale bar, 22 μm). (i–k) Lymphoma sections from the mesenteric lymph node of anNDRG2+/−mouse. The histopathology indicated the presence of diffuse pleomorphic large lymphoid cells with vesicular nuclei, prominent nucleoli and scant cytoplasm (i). Robust staining for CD3 was present in the cytoplasm (j), but B220 staining was negative (k) (scale bar, 22 μm). (l–n) Lymphoma sections from anNDRG2+/−mouse spleen were examined by histopathology. The results demonstrated pleomorphic large lymphoid cells with vesicular nuclei, prominent nucleoli, some nuclear distortion and numerous cells undergoing mitosis (l). Staining for CD3 revealed robust cytoplasmic staining in cells, ranging from white pulp to red pulp (m). B220 staining was negative (n) (scale bar, 22 μm). 6f ), and they developed various types of tumours, including lymphoma, hepatocellular carcinoma and bronchoalveolar carcinoma ( Supplementary Table 6 ; Fig. 6g,h ). Malignant lymphomas occurred at a high frequency (~50%), and the infiltrating lymphoid cells were CD3 + CD4 + CD8 − , indicating a mature helper T-cell phenotype ( Fig. 6i–n ; Supplementary Fig. 21 ), suggesting that NDRG2 is a possible tumour suppressor in various types of cancer, including peripheral T-cell lymphoma. Figure 6: NDRG2 -deficient mice are susceptible to tumour formation. ( a ) Western blots of 3-month-old adult tissues of WT mice. The data are representative of two experiments. ( b ) Western blots of various tissues of 3-month-old NDRG2 -deficient mice. The data are representative of two experiments. ( c ) The co-immunoprecipitation of PTEN and NDRG2 in frontal cortex homogenates from 3-month-old WT mice. The data are representative of three experiments. ( d ) Whole-cell lysates from WT, NDRG2 +/− and NDRG2 −/− embryonic fibroblasts were subjected to western blotting. ( e ) The proliferation rates of WT, NDRG2 +/− , and NDRG2 −/− embryonic fibroblasts. The mean±s.d. is shown; * P <0.05 (Student’s t- test). The data are representative of three experiments. ( f ) Kaplan–Meier survival curves of WT ( n =15), NDRG2 +/− ( n =31) and NDRG2 −/− ( n =12) mice up to 24 months of age. The difference in survival was statistically significant between WT and NDRG2 +/− or NDRG2 −/− mice (* P <0.05, log-rank test). ( g ) A hepatocellular carcinoma section from an NDRG2 +/− mouse liver was subjected to H&E staining. The results indicated the presence of a large sheet of hepatic cords composed of several hepatocytes of variable nuclei and cell sizes; the nuclei of the carcinoma cells were hyperchromatic with prominent nucleoli (scale bar, 22 μm). ( h ) A bronchoalveolar carcinoma section from an NDRG2 +/− mouse lung was subjected to H&E staining. The histopathology demonstrated a well-circumscribed mass of a solid sheet of neoplastic cells containing hyperchromatic nuclei with signs of frequent mitosis and an indistinct basophilic cytoplasm (scale bar, 22 μm). ( i – k ) Lymphoma sections from the mesenteric lymph node of an NDRG2 +/− mouse. The histopathology indicated the presence of diffuse pleomorphic large lymphoid cells with vesicular nuclei, prominent nucleoli and scant cytoplasm ( i ). Robust staining for CD3 was present in the cytoplasm ( j ), but B220 staining was negative ( k ) (scale bar, 22 μm). ( l – n ) Lymphoma sections from an NDRG2 +/− mouse spleen were examined by histopathology. The results demonstrated pleomorphic large lymphoid cells with vesicular nuclei, prominent nucleoli, some nuclear distortion and numerous cells undergoing mitosis ( l ). Staining for CD3 revealed robust cytoplasmic staining in cells, ranging from white pulp to red pulp ( m ). B220 staining was negative ( n ) (scale bar, 22 μm). Full size image NDRG2 downregulation activates PI3K-AKT in various cancers We next evaluated the methylation status of the NDRG2 promoter in various cancer cell lines from different organ origins. 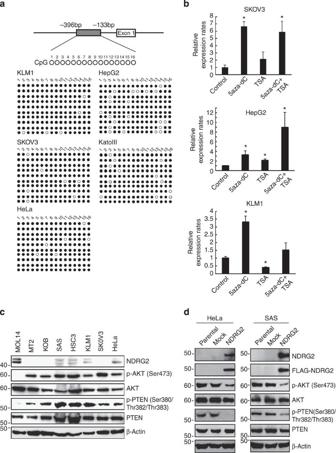Figure 7: Downregulation ofNDRG2is associated with enhanced phosphorylation of PTEN-Ser380/Thr382/Thr383 and enhanced activation of PI3K-AKT in various cancers. (a) Bisulfite genomic sequencing of theNDRG2promoter region in the KLM1 (pancreatic cancer), SKOV3 (ovarian cancer), HeLa (cervical cancer), HepG2 (hepatic cancer) and KatoIII (gastric cancer) cell lines. PCR products amplified from bisulfite-treated genomic DNA were subcloned, and ten clones in each cell line were sequenced. Open circles indicate unmethylated CpGs (Thy) and filled circles indicate methylated CpGs (Cyt). The region sequenced spans from −396 bp to −133 bp. (b) SKOV3, HepG2 and KLM1 cells were cultured with 10 μM 5-aza-dC for 72 h, with 1.2 μM TSA for 48 h, or with 1.2 μM of TSA for 48 h, followed by 10 μM of 5-aza-dC for 24 h. After treatments, total RNA was extracted and quantitative RT–PCR was performed withNDRG2and β-actin. The relative amounts of mRNA were normalized against β-actin mRNA and expressed relative to the mRNA abundance in untreated cells. The mean±s.d. is shown; *P<0.05 compared with the untreated control (Student’st-test). The data are representative of two experiments. (c) Western blot analyses of NDRG2, PTEN, p-PTEN (Ser380/Thr382/Thr383), AKT and p-AKT (Ser473) were performed in SAS (OSCC), HSC3 (OSCC), KLM1, SKOV3, HeLa, MT2 (ATLL), KOB (ATLL) and MOLT4 (T-ALL) cell lines. The data are representative of two experiments. (d) HeLa and SAS cells stably transfected with Mock or FLAG-NDRG2 expression vector were subjected to western blotting. The data are representative of three experiments. In accordance with previous studies [30] , [31] , methylation of the NDRG2 promoter was found in various cancer types ( Supplementary Table 7 ; Fig. 7a ). We confirmed that treatment of these cancer cell lines with 5-aza-deoxycytidine resulted in an increased abundance of NDRG2 mRNA ( Fig. 7b ). Recently, we reported that the abundance of phosphorylated AKT-Ser473 inversely correlated well with NDRG2 protein abundance in the majority of oral squamous cell carcinoma (OSCC) cases [32] , which are known to have very low frequencies of PTEN and PIK3CA mutations [33] , [34] . We found that cancer cell lines with low levels of NDRG2 show high levels of phosphorylated PTEN-Ser380/Thr382/Thr383 and AKT-Ser473 ( Fig. 7c ). Of note, we found that the ectopic expression of NDRG2 in two human cancer cell lines carrying WT PTEN ((SAS (OSCC) and HeLa (cervical cancer)) resulted in marked decreases in PTEN-Ser380/Thr382/Thr383 phosphorylation and PI3K-AKT inactivation ( Fig. 7d ). These findings suggest that downregulation of NDRG2 could have an important role in activating the PI3K-AKT signalling pathway in various types of cancer. Figure 7: Downregulation of NDRG2 is associated with enhanced phosphorylation of PTEN-Ser380/Thr382/Thr383 and enhanced activation of PI3K-AKT in various cancers. ( a ) Bisulfite genomic sequencing of the NDRG2 promoter region in the KLM1 (pancreatic cancer), SKOV3 (ovarian cancer), HeLa (cervical cancer), HepG2 (hepatic cancer) and KatoIII (gastric cancer) cell lines. PCR products amplified from bisulfite-treated genomic DNA were subcloned, and ten clones in each cell line were sequenced. Open circles indicate unmethylated CpGs (Thy) and filled circles indicate methylated CpGs (Cyt). The region sequenced spans from −396 bp to −133 bp. ( b ) SKOV3, HepG2 and KLM1 cells were cultured with 10 μM 5-aza-dC for 72 h, with 1.2 μM TSA for 48 h, or with 1.2 μM of TSA for 48 h, followed by 10 μM of 5-aza-dC for 24 h. After treatments, total RNA was extracted and quantitative RT–PCR was performed with NDRG2 and β-actin. The relative amounts of mRNA were normalized against β-actin mRNA and expressed relative to the mRNA abundance in untreated cells. The mean±s.d. is shown; * P <0.05 compared with the untreated control (Student’s t- test). The data are representative of two experiments. ( c ) Western blot analyses of NDRG2, PTEN, p-PTEN (Ser380/Thr382/Thr383), AKT and p-AKT (Ser473) were performed in SAS (OSCC), HSC3 (OSCC), KLM1, SKOV3, HeLa, MT2 (ATLL), KOB (ATLL) and MOLT4 (T-ALL) cell lines. The data are representative of two experiments. ( d ) HeLa and SAS cells stably transfected with Mock or FLAG-NDRG2 expression vector were subjected to western blotting. The data are representative of three experiments. Full size image In this study, we show that NDRG2 interacts with PTEN and promotes its dephosphorylation at Ser380/Thr382/Thr383 by recruiting PP2A to PTEN. We also demonstrated that loss of NDRG2 expression via genetic or epigenetic abnormalities in ATLL cells can contribute to the increase in PTEN-Ser380/Thr382/Thr383 phosphorylation, which leads to inactivation of PTEN lipid phosphatase activity and activation of the PI3K-AKT pathway. The imbalance of the expression of NDRG2 and as yet unidentified protein kinases might account for an elevation of PTEN-Ser380/Thr382/Thr383 phosphorylation with a high amount of phosphorylated AKT in ATLL cells. Finally, we showed that NDRG2- deficient mice develop multiple types of tumours, thus establishing that loss of NDRG2 expression can contribute to tumour development. PTEN stability and lipid phosphatase activity can be regulated through phosphorylation of the C-terminal tail, which contains a cluster of serine–threonine residues: Ser370, Ser380, Thr382, Thr383 and Ser385 (ref. 35 ). Although the cluster of Ser380/Thr382/Thr383 residues in the C-terminal tail are thought to be minor phosphorylation sites [26] , [36] , the level of phosphorylated PTEN-Ser380/Thr382/Thr383 has been shown to be rapidly and transiently increased in hypothalamic cells treated with leptin and in rat brains following transient middle cerebral artery occlusion [37] , [38] . CK2 is known to be a major kinase that phosphorylates PTEN at the C-terminal serine–threonine cluster, but phosphorylation of Ser380/Thr382/Thr383 by CK2 is still under debate [21] , [26] , [36] , [39] . We observed that suppression of CK2 activity with specific inhibitors in ATLL cells did not influence PTEN-Ser380/Thr382/Thr383 phosphorylation. Thus, it is likely that CK2 is not responsible for the phosphorylation of PTEN at Ser380/Thr382/Thr383 in ATLL cells. In contrast, the expression of NDRG2 is markedly upregulated in several tumour cell lines exposed to hypoxic conditions and is thought to be a new hypoxia-inducible factor-1 target gene [40] , [41] . It could be speculated that NDRG2 expression is induced by hypoxia-ischemia in the brain to regulate PTEN phosphorylation, leading to the suppression of PI3K-AKT activation and induction of apoptosis. Interestingly, several kinases, including SGK1 (serum- and glucocorticoid-induced kinase 1), PKCθ (protein kinase C-θ) and AKT, have been found to phosphorylate NDRG2 (refs 42 , 43 ). These phosphorylation events are likely to affect the cellular function of NDRG2. It is intriguing to speculate that NDRG2 might be a downstream target of the PI3K-AKT signalling pathway that may participate in a negative feedback loop in PI3K-AKT signalling. PP2A exists predominantly as a heterotrimer composed of catalytic C, structural A and one member of four families of regulatory B subunits. The activity, substrate specificity and subcellular localization of the PP2A holoenzyme are thought to be determined by its B subunit [44] . A recent study has shown that following AKT phosphorylation, Clk2 is activated and phosphorylates the PP2A regulatory subunit B56β, thereby leading to the assembly of the PP2A holoenzyme complex on AKT and dephosphorylation of AKT at both Thr308 and Ser473 (ref. 45 ). Thus, a more complex feedback regulation governing NDRG2 and PP2A activities may exist within the PI3K-AKT pathway. Identifying the PP2A regulatory subunit that interacts with NDRG2 would provide important clues in understanding how the dephosphorylation of PTEN by NDRG2-PP2A is regulated upon AKT activation. Elevated phosphorylation of PTEN-Ser380/Thr382/Thr383 with high levels of activated AKT is frequently observed in acute myeloid leukaemia (AML) and is associated with poor prognosis [46] . The phosphorylation of Ser380/Thr382/Thr383 is also elevated in human fibromyomatous uteri and may be a contributory factor in the development of uterine leiomyomas [47] . Although it is not known whether these phosphorylation events are attributed to the functional inactivation of NDRG2 , decreased expression and promoter methylation of the NDRG2 gene have been reported in various types of cancer, such as liver cancers, gastric cancers, colon cancers and glioblastomas [30] , [31] , [48] , [49] , [50] , [51] . Therefore, we hypothesize that in ATLL and other types of tumour cells without genetic alterations in the PI3K-AKT pathway, the suppression of NDRG2 transcription disrupts the negative regulation of PI3K-AKT signalling via sustained PTEN-Ser380/Thr382/Thr383 phosphorylation during tumour development ( Fig. 8 ). The finding that PTEN-Ser380/Thr382/Thr383 is highly phosphorylated in all of the organs of NDRG2 -deficient mice provides additional evidence that the balance between an unidentified PTEN-Ser380/Thr382/Thr383 kinase(s) and PP2A-NDRG2 activity regulates the phosphorylation status of PTEN-Ser380/Thr382/Thr383 in vivo . Therefore, we are currently attempting to identify the protein kinase(s) that target PTEN-Ser380/Thr382/Thr383, which has the potential to be a therapeutic drug target in a variety of cancers, including ATLL. 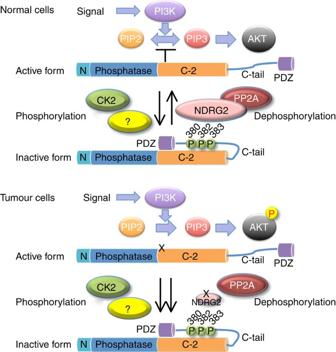Figure 8: Schematic model for the regulation of PTEN activity by NDRG2. In normal cells, PP2A is efficiently recruited to PTEN via its interaction with NDRG2, which may facilitate dephosphorylation of PTEN at Ser380/Thr382/Thr383, resulting in an active open conformation of PTEN and subsequently leading to the dephosphorylation of PIP3to PIP2. In tumour cells, expression of NDRG2 is inhibited by DNA methylation of its promoter, causing sustained phosphorylation of PTEN, which keeps PTEN in an inactive closed conformation. Loss of PTEN activity leads to increased PIP3levels and AKT activation. The balance between the expression of NDRG2 and an unidentified kinase(s) may have an important role in regulating the phosphorylation status of PTEN. Figure 8: Schematic model for the regulation of PTEN activity by NDRG2. In normal cells, PP2A is efficiently recruited to PTEN via its interaction with NDRG2, which may facilitate dephosphorylation of PTEN at Ser380/Thr382/Thr383, resulting in an active open conformation of PTEN and subsequently leading to the dephosphorylation of PIP 3 to PIP 2 . In tumour cells, expression of NDRG2 is inhibited by DNA methylation of its promoter, causing sustained phosphorylation of PTEN, which keeps PTEN in an inactive closed conformation. Loss of PTEN activity leads to increased PIP 3 levels and AKT activation. The balance between the expression of NDRG2 and an unidentified kinase(s) may have an important role in regulating the phosphorylation status of PTEN. Full size image Because NDRG2 has been shown to have growth inhibitory effects on several malignant cell lines through downregulation of several signalling pathways, including PI3K-AKT, janus kinase-signal transducer and activator of transcription (JAK-STAT) and nuclear factor-kappaB signalling [52] , [53] , one may speculate that the phosphorylation of different proteins involved in these signalling pathways is regulated by the PP2A-NDRG2 complex. Indeed, we observed that the ectopic expression of NDRG2 in ATLL cells causes suppression of JAK-STAT and nuclear factor-kappaB activation (data not shown), although the molecular mechanisms underlying these effects are still being elucidated. We speculate that NDRG2 may have a key role in suppressing different oncogenic signalling pathways in tumourigenesis. In conclusion, this study provides the first functional evidence for a tumour suppressor role of NDRG2 and suggests that NDRG2 is involved in the leukaemogenesis of ATLL. Further investigations of the roles of NDRG2 in the regulation of different signalling pathways may provide clues in understanding the underlying mechanisms of cancer. Cell lines Jurkat, MOLT4, KAWAI and MKB1 are HTLV-1-negative human T-ALL cell lines. KOB, SO4 and KK1 are IL2-dependent ATLL cell lines. ED, Su9T-01 and S1T are IL2-independent ATLL cell lines. MT2, MT4 and HUT102 are human T-cell lines transformed by HTLV-1 infection. Jurkat, MOLT4 and MKB1 were obtained from the Fujisaki Cell Center, Hayashibara Biochemical Laboratories (Okayama, Japan). KAWAI was kindly provided by Dr Y. Hayashi (Gunma Children's Medical Center, Gunma, Japan). MT2, MT4 and HUT102 were kind gifts from Dr H. Iha (Oita University, Oita, Japan). KOB, SO4 and KK1 were kind gifts from Dr Y. Yamada (Nagasaki University, Nagasaki, Japan). Su9T-01 and S1T were kind gifts from Dr N. Arima (Kagoshima University, Kagoshima, Japan). ED was a kind gift from Dr M. Maeda (Kyoto University, Kyoto, Japan). AML cell lines UCSD/AML1, Kasumi-3, K051, NH and MOLM1 were obtained from Dr R. Taetle (VA Medical Center, Sepulveda, CA, USA), from Dr H. Asoh (Hiroshima University, Hiroshima, Japan), from Dr T. Nomura (Nippon Medical School, Tokyo, Japan), from Dr K. Suzukawa (University of Tsukuba, Ibaraki, Japan) and from the Fujisaki Cell Center, Hayashibara Biochemical Laboratories (Okayama, Japan), respectively, and OIH-1 and FKH-1 were obtained from Dr H. Hamaguchi (Musashino Red Cross Hospital). Pancreatic cancer cell lines KLM1, PK9 and PK45P, OSCC cell lines SAS, HO-1-U-1, Ca9-22, HSC2, HSC3, HSC4, HSQ89 and Sa3, cervical cancer cell line HeLa, human embryonic kidney cell line HEK293T and mouse embryonic fibroblast cell line NIH3T3 were obtained from RIKEN Bioresource Center (Tsukuba, Japan). Hepatic cancer cell lines HLF and HuH28 and breast cancer cell line SK-BR-3 were obtained from the Japanese Cancer Research Resources Bank (Tokyo, Japan). Hepatic cancer cell lines HepG2 and HuH7 were obtained from the Health Science Research Resources Bank (Osaka, Japan). Lung cancer cell lines A549, H322, H1395, H1437 and H1648 were obtained from the American Type Culture Collection (Rockville, MD, USA). Glioblastoma cell line A172 and neuroblastoma cell lines NH6 and NH12 were kind gifts from Dr Y. Hayashi (Gunma Children's Medical Center, Gunma, Japan). Prostate cancer cell line PC3 was a kind gift from Dr T. Ochiya (National Cancer Center Research Institute, Tokyo, Japan). Gastric cancer cell lines Mkb28, Mkb45, and KatoIII and ovarian cancer cell line SKOV3 were kind gifts from Dr H. Kataoka (University of Miyazaki, Miyazaki, Japan). IL2-dependent ATLL cell lines were maintained in RPMI 1640 medium (Wako) supplemented with 10% fetal bovine serum and 50 JRU per ml recombinant human IL2 (Takeda). HTLV-1-negative cell lines, cell lines transformed with HTLV-1 and IL2-independent ATLL cell lines were maintained in the same medium without IL2. The other cell lines were cultured in RPMI 1640 or Dulbecco's modified Eagle's medium (Wako) supplemented with 10% fetal bovine serum. Patient samples Blood samples were obtained with informed consent with approval by the Institutional Review Board of the Faculty of Medicine, University of Miyazaki. ATLL cells were collected from the patients at the time of hospital admission before the chemotherapy started. The diagnosis of ATLL was based on clinical features, hematological characteristics and the presence of anti-HTLV-1 antibodies in the sera. Monoclonal HTLV-1 provirus integration into the DNA of leukaemic cells was confirmed by Southern blot analysis in all cases. Peripheral blood mononuclear cells (PBMCs) obtained from healthy volunteers and patients with ATLL were purified by gradient centrifugation (Sigma-Aldrich). The procedure for the isolation of ATLL cells from PBMCs has been described elsewhere [54] . CD4 + T cells were purified from PBMCs of healthy volunteers by using anti-CD4 magnetic beads (Miltenyi Biotec) according to the manufacturer's instructions. Antibodies and reagents A synthetic peptide (17-PGQTPEAAKTHSVET-31) of human NDRG2 conjugated to keyhole limpet haemocyanin was used for immunization to generate a rabbit polyclonal antibody against NDRG2 (ref. 55 ). Mouse monoclonal (M2) and rabbit polyclonal (F7425) antibodies against FLAG, and mouse monoclonal antibody (AC-15) against β-actin were purchased from Sigma-Aldrich. Rabbit monoclonal antibodies against PTEN (138G6), phospho-AKT (Ser473) (D9E), phospho-AKT (Thr308) (244F9), phospho-GSK3β (Ser9) (D85E12), GSK3β (27C10), and PP2A C Subunit (PP2Ac) (52F8), rabbit polyclonal antibodies against phospho-PTEN (Ser380/Thr382/383) (9554), non-phospho-PTEN (Ser380/Thr382/383) (9569), AKT (9272), FOXO1/4 (9462) and cleaved caspase-3 (9661), and mouse monoclonal antibodies against PTEN (26H9) and Myc-tag (9B11) were obtained from Cell Signaling Technology. Rabbit polyclonal antibodies against phospho-PTEN (Ser370) (07-889) and PI3K p85 (06-195) were obtained from Upstate/Millipore, rabbit polyclonal antibody against phospho-PTEN (Ser385) (44-1064G) was obtained from Biosource, mouse monoclonal antibody against SHIP1 (P1C1) and goat polyclonal antibody against NDRG2 (E20) were obtained from Santa Cruz Biotechnology, rabbit polyclonal antibody against GFP (598) was obtained from MBL, and rat monoclonal antibodies against mouse B220 (RA3-6B2), mouse CD4 (RM4-5) and mouse CD8 (53-6.7) and hamster monoclonal antibody against mouse CD3 (500A2) were obtained from BD Pharmingen. Mouse monoclonal antibody against TAX (MI73) was a kind gift from Dr M. Matsuoka (Kyoto University, Kyoto, Japan). Recombinant human PP2A core enzyme made up of polyhistidine-tagged (His 8X ) human PP2Ac and FLAG-tagged human PR65/A co-expressed in baculovirus-infected High Five cell, OA and trichostatin A were obtained from Wako. Dimethyl 3,3′-dithiobispropionimidate (DTBP) was obtained from Thermo Fisher Scientific, and TBB was obtained from Calbiochem. CX-4945 was obtained from Selleckchem, and 5-aza-2’-deoxycytidine was obtained from Sigma-Aldrich. Plasmid construction Full-length complementary DNA (cDNA) of NDRG2 was isolated by RT–PCR from total RNA of the MOLT4 cell line and subcloned into the p3XFLAG-myc-CMV-26 expression vector (Sigma-Aldrich) by standard cloning procedures (FLAG-NDRG2). The FLAG-tagged NDRG2 deletion constructs—NDRG2-deltaN (amino acids 26–357), NDRG2-deltaC (amino acids 1–304), NDRG2-NDR (amino acids 26–304), NDRG2-HD (amino acids 81–297) and NDRG2-Cterm (amino acids 259–357)—were generated by PCR using the NDRG2/pCMV26 as the template and subcloned into p3XFLAG-myc-CMV-26. The GFP-PTEN constructs—GFP-PTEN, GFP-PTEN-N (amino acids 1–185) and GFP-PTEN-C (amino acids 186–403)—were generated by PCR using the PTEN/pcDNA3 (a kind gift from Dr T. Kohno, National Cancer Center Research Institute, Tokyo, Japan) as the template and subcloned into pEGFP-C1 vector (Clontech). A full-length PTEN cDNA was amplified from the Su9T-01 cell line by PCR and subcloned into the p3XFLAG-myc-CMV-26. To generate substitution mutant PTEN expression vectors (PTEN-S370A, -S380A/T382A/T383A and -S385A), PCR-based mutagenesis were performed to introduce mutations in the PTEN coding sequence using mutagenic primers listed in Supplementary Table 8 and p3XFLAG-myc-CMV-26/PTEN plasmid as the template. All PCR-generated products were confirmed by nucleotide sequencing. The expression vector for constitutively active PI3K (pmycBD110) [56] , which carries the p110-binding domain of p85α attached to the N-terminal region of p110, was kindly provided by Dr Y. Fukui (National Health Research Institutes, Taiwan). The myc-PP1c/pcDNA3, myc-PP2Ac/pcDNA3 and myc-PP5c/pcDNA3 constructs have been described elsewhere [57] . Bisulfite sequencing A 200-ng DNA sample was denatured in 0.2 M NaOH followed by the addition of bisulfite solution (2.5 M sodium bisulfite, 10 mM hydroquinone and 240 mM NaOH). The mixture was then incubated at 55 °C for 16 h. DNA samples were desulfonated in 0.2 M NaOH and precipitated with ethanol. PCR was performed in a 20-μl volume containing 1 μl of bisulfite-treated DNA, 500 μM of dNTP and 500 nM of each primer for the NDRG2 promoter region (nucleotides 20564110-20563790, GenBank accession no. NC_000014) (forward 5′-TTTTCGAGGGGTATAAGGAGAGTTTATTTT-3′ and reverse 5′-CCAAAAACTCTAACTCCTAAATAAACA-3′) (ref. 48 ), and 1 unit of Taq polymerase (Takara) under the following conditions: 98 °C for 30 s; 40 cycles of 98 °C for 10 s, 60 °C for 5 s and 72 °C for 30 s; and final extension at 72 °C for 3 min. PCR products were subcloned into the pTA2 vector (TOYOBO) and sequenced. Real-time RT–PCR analysis Total RNA was isolated from cells using TRIzol reagent (Invitrogen) and 1 μg of total RNA was reverse transcribed to obtain first-strand cDNA using an RNA-PCR kit (Takara) following the manufacturer's instructions. The resulting cDNA was used for real-time RT–PCR using a SYBR Green PCR Master Mix kit (Applied Biosystems). PCR was performed in a 25-μl volume containing 1 μl cDNA, 300 μM of each primer and 12.5 μl of 2 × PCR master mix under the following conditions: 95 °C for 10 min followed by 40 cycles of 95 °C for 15 s and 60 °C for 1 min. For NDRG2 primers, the cycling conditions were 95 °C for 10 min, 40 cycles of 95 °C for 15 s, 60 °C for 20 s and 72 °C for 40 s. The primers used were as follows: for PTEN , PTEN-F (5′-CAGCCATCATCAAAGAGATCG-3′) and PTEN-R (5′-TTGTTCCTGTATACGCCTTCAA-3′); for NDRG2 , NDRG2-F (5′-CTGGAACAGCTACAACAACC-3′), and NDRG2-R (5′-TCAACAGGAGACCTCCATGG-3′); and for β-actin, ACTB-F (5′-GACAGGATGCAGAAGGAGATTACT-3′), and ACTB-R (5′-TGATCCACATCTGCTGGAAGGT-3′). The data were normalized to the amount of β-actin mRNA, and the values are represented as the mean±s.d. of 2 −ΔΔCt in a duplicate assay. Western blot analysis Cell lysate samples were prepared in NP-40 lysis buffer (50 mM Tris–HCl, pH 8.0, 150 mM NaCl, 5 mM EDTA, 1% NP-40) supplemented with protease inhibitor cocktail (Sigma-Aldrich) and phosphatase inhibitors (PhosStop, Roche) or by direct lysis in boiling Laemmli SDS sample buffer (62.5 mM Tris–HCl, pH 6.8, 2% SDS, 25% glycerol, 5% β-mercaptoethanol and 0.01% bromophenol blue). Protein samples were electrophoresed on 10% SDS-polyacrylamide gel and transferred to polyvinylidine difluoride membranes (Immobilon-P, Millipore). The membranes were blocked in Tris-buffered saline (TBS)-Tween (0.1%) with either 5% bovine serum albumin (BSA) or 5% nonfat dried milk and were then incubated with each primary antibody diluted in TBS containing 0.1% Tween 20 supplemented with either 5% nonfat dried milk or 5% BSA or in the Can Get Signal buffer (TOYOBO). Bound antibody was detected by a Lumi-light Plus kit according to the manufacturer’s instructions (Roche Diagnostics). Band intensities on blots were quantified using NIH Image J software. All primary antibodies were used at a dilution of 1:1,000, except anti-β-actin (1:5,000) and anti-NDRG2 (E20, 1:250). Representative full-gel bots are provided in the Supplementary Fig. 22 ) Immunoprecipitation assays For detecting interaction between endogenous proteins, MOLT4 cells (1 × 10 7 ) and mouse frontal cortex tissue were solubilized with RIPA buffer (50 mM Tris–HCl, pH 7.8, 150 mM NaCl, 1% NP-40, 0.25% sodium deoxycholate and 1 mM EDTA) and NP-40 lysis buffer, respectively, supplemented with protease inhibitor cocktail (Sigma-Aldrich) and phosphatase inhibitors (PhosStop, Roche), and the lysates were then incubated with control rabbit immunoglobulin G or antibodies against NDRG2 (rabbit polyclonal, 1:500 or E20, 1:200) or PTEN (26H9, 1:100 or 138G6, 1:300), plus Protein G beads (Amersham Biosciences). After washing, the bound proteins were subjected to SDS-polyacrylamide gel electrophoresis (SDS-PAGE) and immunoblotting with antibodies against NDRG2 (rabbit polyclonal or E20) or PTEN (26H9 or 138G6). For overexpressed proteins, 293T cells were co-transfected with the indicated constructs using HilyMax (Dojindo) according to the manufacturer’s instructions. After culturing for 48 h, the transfected cells were solubilized with RIPA buffer, and the lysates were then subjected to immunoprecipitation using FLAG M2 affinity gel (Sigma-Aldrich) or antibodies against GFP (1:200) or PTEN (138G6, 1:500), followed by immunoblotting with antibodies against either FLAG (F7425), GFP or PTEN (26H9). For chemical crosslinking, stable HUT102 or KK1 cell lines expressing FLAG-NDRG2 were washed twice with phosphate-buffered saline (PBS) and incubated with 2 mM DTBP in PBS at room temperature for 30 min. After washing twice with PBS, cells were lysed in TNT buffer (10 mM Tris–HCl, pH 7.5, 150 mM NaCl and 0.5% Triton X-100) supplemented with protease inhibitor cocktail (Sigma-Aldrich) and phosphatase inhibitors (Halt phosphatase inhibitor cocktail, Thermo Scientific), and the lysates were immunoprecipitated with control rabbit immunoglobulin G, antibody against PTEN (138G6, 1:500), or FLAG M2 affinity gel, followed by immunoblotting with antibodies against FLAG (F7425), PP2Ac, PTEN (138G6) or phospho-PTEN (Ser380/Thr382/Thr383). Immunofluorescence staining Cells were fixed with 4% paraformaldehyde for 10 min at room temperature, washed with TBS 0.1 M glycine, treated with 0.2% Triton X-100 and rewashed with TBS 0.1 M glycine. After blocking with 1% BSA in TBS, cells were incubated with primary antibodies against NDRG2 (E20, 1:100), FoxO1/4 (1:200), PTEN (138G6, 1:200) or FLAG (M2, 1:500) overnight at 4 °C. The cells were then washed three times with TBS containing 0.1% Tween 20 and incubated with Alexa Fluor-546 anti-mouse, Alexa Fluor-555 anti-rabbit, Alexa Fluor-488 anti-rabbit or Alexa Fluor-488 anti-goat secondary antibodies (Molecular Probes) at room temperature for 2 h. The coverslips were washed three times with TBS containing 0.1% Tween 20 and then mounted on glass slides using an antifade reagent (Invitrogen). Proteins were visualized using a confocal laser scanning microscope (Leica Microsystems). Nuclei were counterstained with 4',6-Diamidino-2-phenylindole (DAPI; Sigma-Aldrich). RNAi treatment DNA-based shRNA expression vector (RNAi-Ready pSIREN-RetroQ-ZsGreen vector, Clontech) and siRNA oligonucleotides were used in gene knockdown experiments. The shRNA target sequences were as follows: for human NDRG2 , shNDRG2#1 (5′-GGTGGAGAGGGCATATGCA-3′) and shNDRG2#2 (5′-GCGAGTCTGGAACTCTTTCTT-3′); for mouse NDRG2 , 5′-CCGTGAAGAACAGTGGTAA-3′. A control shRNA vector targeting luciferase (shLuc) was purchased from Clontech. The PP2Acα siRNA (sc-43509) and control siRNA (6568) were purchased from Santa Cruz Biotechnology and Cell Signaling Technology, respectively. The transfections were performed using the Nucleofector V kit (Amaxa) following the company's protocol. Cell proliferation assays Cells were seeded onto 96-well microtiter plates at a density of 5 × 10 3 per well and cultured for the indicated time periods. Viable cells were counted by the methyl thiazolyl tetrazolium assay using a cell counting kit-8 (Dojindo). For stable transfectant cells, cells were seeded into 25 cm 2 flasks at a density of 1 × 10 5 ml −1 , and proliferation rates were assessed by counting the numbers of viable cells every 24 h using Trypan blue staining. Dephosphorylation assay for synthetic peptides The PTEN peptide 373-EPDHYRYSDTTDSDPENE-390 and phosphopeptides with pSer380 (EPDHYRYpSDTTDSDPENE), pThr382 (EPDHYRYSDpTTDSDPENE), pThr383 (EPDHYRYSDTpTDSDPENE) and pSer380/pThr382/pThr383 (EPDHYRYpSDpTpTDSDPENE) were obtained from TORAY Research Center (Tokyo, Japan). The release of inorganic phosphates from phosphopeptides was determined using a malachite green assay kit (BIOMOL Green reagent, BIOMOL). Cell extracts from the KK1-NDRG2 stable cell line, NIH3T3 cell line and 293T cell line transiently transfected with mock or Myc-tagged PP1c, PP2Ac or PP5c vectors using HilyMax were prepared by lysing cells in TNT buffer supplemented with protease inhibitor cocktail (Sigma-Aldrich). Endogenous PP2Ac and Myc-tagged PP1c, PP2Ac and PP5c were immunoprecipitated using antibodies against anti-PP2Ac (1:500) and anti-Myc (1:500), respectively. For inhibitor treatment, lysates of KK1-NDRG2 cells were incubated on ice for 30 min in the absence or presence of various concentrations of OA. The total cell lysates, immunoprecipitated samples or 0.5 units of recombinant PP2A were incubated with 100 μM PTEN peptide or phosphopeptides in 10 μl of phophatase assay buffer (20 mM HEPES pH 7.0, 1 mM MnCl 2 , 8 mM MgCl 2 , 1 mM dithiothreitol and 100 μg ml −1 BSA) at 30 °C for 60 min. The reactions were terminated by the addition of 40 μl of TE buffer (10 mM Tris–HCl, pH 8.0, 1 mM EDTA) and 100 μl of BIOMOL Green reagent, and absorbance at 620 nm was determined after incubation for 20 min at room temperature. The quantity of Pi released (nmoles) was calculated based on a standard curve determined for inorganic phosphate according to the manufacturer’s recommendations. All assays were performed in duplicate. PTEN dephosphorylation assay The KK1-Mock stable cells were lysed in TNT buffer plus protease inhibitor cocktail (Sigma-Aldrich), and the cell lysates were immunoprecipitated with an antibody against PTEN (138G6, 1:500) and Protein G beads. Immunoprecipitates were washed three times with TNT buffer and twice with phosphatase assay buffer, resuspended in phosphatase assay buffer and incubated with 0.5 units of recombinant PP2A for 60 min at 30 °C. The reaction was stopped by adding SDS sample buffer, and the samples were separated by 10% SDS-PAGE, followed by western blotting with antibodies against PTEN (138G6) or phospho-PTEN (Ser370 or Ser380/Thr382/Thr383). Generation of NDRG2 knockout mice NDRG2 -deficient mice were generated in the Laboratory for Animal Resources and Genetic Engineering, RIKEN Center for Developmental Biology (accession. no. CDB0768K: http://www.cdb.riken.jp/arg/mutant%20mice%20list.html ). For generating a targeting vector, genomic fragments for NDRG2 were obtained from RP23-109J8 BAC clone (BACPAC Resources). A lacZ -pA- neo -pA cassette was inserted into exon 2 of the NDRG2 gene to create the targeting construct. The linearized targeting vector was inserted into TT2 ES cells [58] by electroporation, and G418-resistant clones were screened for homologous recombination by PCR and Southern blot analysis using a 457-bp 5′ fragment as the probe. Targeted ES clones were microinjected into ICR eight-cell stage embryos and transferred into pseudopregnant ICR females ( http://www.cdb.riken.jp/arg/Methods.html ). The resulting chimeras were bred with C57BL/6 mice, and heterozygous offspring were identified by Southern blot analysis and by PCR using the following two primer pairs: WT allele, F1 (5′-CAAACACCCGAGACTGCCAA-3′)/R (5′-ATTAAACAATAAAGATGTCC-3′); targeted-allele, F2 (5′-GACAGGAGAGGATGAAGGTT-3′)/R. Heterozygous mice were backcrossed with C57BL/6 for two generations and mated in the same generation to obtain homozygous mutants. All animal experiments were approved by the Animal Experiment Review Board of the University of Miyazaki. Histological analysis All necropsies and histological examinations were performed on mice at the time of death. Tissues were fixed in 10% buffered formalin solution and embedded in paraffin blocks, and 2-μm-thick sections were prepared. Paraffinized sections were deparaffinized with xylene and rehydrated through a decreasing gradient of ethanol solutions. Slides were stained with hematoxylin and eosin (H&E), coverslipped with mounting medium, and viewed under a light microscope. The slides were scanned with a digital scanner (MIRAX; Carl Zeiss) and viewed with MIRAX software (Carl Zeiss). For immunohistochemistry, the tissue sections were deparaffinized and rehydrated. After microwave treatment for 20 min in citrate buffer pH 6.0 and cooling, endogenous peroxidase activity was blocked in 0.3% hydrogen peroxide in methanol for 30 min. After blocking in 5% skim milk in PBS for 30 min, sections were incubated with antibodies against CD3, CD4, CD8, B220, FLAG or cleaved caspase-3 for 60 min at 37 °C, washed three times with PBS and incubated with horseradish peroxidase-conjugated secondary antibodies for 30 min at 37 °C. The horseradish peroxidase activity was visualized with 3, 3′-diaminobenzidine containing hydrogen peroxide. All primary antibodies were used at 1:200 dilution, except anti-FLAG (1:500) and anti-cleaved caspase-3 (1:100). Statistical analysis Bars and markers in the figures represent the mean±s.d. The two-tailed Student’s t- test and Mann–Whitney U -test were used as appropriate. In the Kaplan–Meier survival analysis, the log-rank test was used for analysis. Fisher’s exact analysis was used to determine differences in tumour incidence. Differences were considered significant when the P value was <0.05, as indicated in the text. How to cite this article: Nakahata, S. et al . Loss of NDRG2 expression activates PI3K-AKT signalling via PTEN phosphorylation in ATLL and other cancers. Nat. Commun. 5:3393 doi: 10.1038/ncomms4393 (2014). Accession codes: The gene expression data have been deposited in the Gene Expression Omnibus database under accession code GSE43017 .